Disruption of a proto-planetary disc by the black hole at the milky way centre Recently, an ionized cloud of gas was discovered plunging towards the supermassive black hole, SgrA*, at the centre of the Milky Way. The cloud is being tidally disrupted along its path to closest approach at ∼ 3,100 Schwarzschild radii from the black hole. Here we show that the observed properties of this cloud of gas can naturally be produced by a proto-planetary disc surrounding a low-mass star, which was scattered from the observed ring of young stars orbiting SgrA*. As the young star approaches the black hole, its disc experiences both photoevaporation and tidal disruption, producing a cloud. Our model implies that planets form in the Galactic centre, and that tidal debris from proto-planetary discs can flag low-mass stars, which are otherwise too faint to be detected. Observations of the galactic centre recently yielded a cloud of ionized gas and dust falling inward on a nearly radial orbit [1] . The cloud will reach pericentre in the summer of 2013, approaching our galaxy's central black hole, SgrA*, at a distance of only 270 AU. As this plunge progresses, tidal gravity from the black hole will disrupt the infalling cloud, providing a unique probe of gas flow near SgrA*. The apocentre of the cloud's orbit, at r apo =8,400 AU=0.04 pc from the black hole, coincides with the inner edge of the ring of young stars orbiting SgrA*, and the plane of the cloud's orbit coincides with that of the ring [1] , [2] . The ring's age, estimated from its population of O/WR stars, is ∼ 4–8 Myr (ref. 3 ). At ages ≲ 3 Myr, most low-mass stars host proto-planetary gas discs [4] with radii of order 100 AU (ref. 5 ), and ∼ 1/5 of stars with mass 0.1−1 M ⊙ retain their discs at ages of ∼ 5 Myr (refs 6 , 7 ). Given the black hole mass of M BH =4.3×10 6 M ⊙ (refs 8 , 9 ), the tidal radius around a star of mass m * at a distance r =0.004 pc from SgrA* is d t ∼ r ( m * /3 M BH ) 1/3 ∼ 40 AU( m * / M ⊙ ) 1/3 . A solar mass star could therefore host a stable disc with a radius of d out ∼ d t /3 ∼ 12 AU on a roughly circular orbit near the inner edge of the young stellar ring. Similarly, an M-dwarf with mass m * =0.3 M ⊙ could host a stable disc having radius d out ∼ 8 AU. We suggest that the newly discovered gas cloud [1] surrounds such a star, which was scattered away from its original ring orbit and is currently plunging towards the supermassive black hole ( Fig. 1 ). The star itself is too low mass to be observable, but the debris produced through the disruption of its proto-planetary disc allowed it to be detected. We first calculate the properties of the system at the cloud's observed location and argue that they match the observations—an ionized cloud ∼ 100 AU in radius with density n ∼ 3×10 5 cm −3 , an electron temperature of 10 4 K and a dust temperature of ∼ 550 K, trailed by a stream of gas. We then provide predictions regarding the evolution of the cloud as it approaches pericentre. Finally, we demonstrate that the probability of producing such an object is plausibly high, and we calculate the implied rate of mass deposition by this process within the young stellar ring. 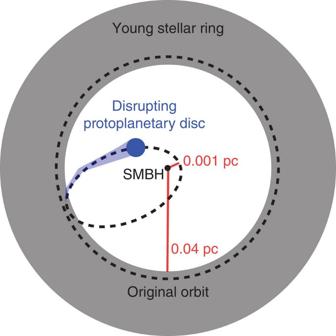Figure 1: Proto-planetary disc plunging towards the galactic centre. Schematic illustration of our scenario. A young, low-mass star hosting a proto-planetary disc is dynamically dislodged from its original orbit (dashed circle) in the Galactic centre's young stellar ring (grey). As it plunges towards the supermassive black hole (SMBH) at the Galactic centre (orbit indicated by dashed ellipse), the disc is photoevaporated and tidally disrupted, generating an extended dusty cloud around the star (blue circle). A trail of dust and gas is deposited along the star's orbit (extended blue trail). Figure 1: Proto-planetary disc plunging towards the galactic centre. Schematic illustration of our scenario. A young, low-mass star hosting a proto-planetary disc is dynamically dislodged from its original orbit (dashed circle) in the Galactic centre's young stellar ring (grey). As it plunges towards the supermassive black hole (SMBH) at the Galactic centre (orbit indicated by dashed ellipse), the disc is photoevaporated and tidally disrupted, generating an extended dusty cloud around the star (blue circle). A trail of dust and gas is deposited along the star's orbit (extended blue trail). Full size image Mass loss Although the tidal radius for a solar-mass star at r =0.04 pc is 40 AU, the tidal radius at the cloud's pericentre distance of r p =270 AU=10 −3 pc is only d t =1 AU ( m * / M ⊙ ) 1/3 . At the most recently observed epoch [1] , the cloud was approximately 6 r p from the black hole, with a tidal radius of 6 AU ( m * / M ⊙ ) 1/3 . Hence, the circumstellar disc is already experiencing substantial tidal disruption. At the same time, the Galactic centre hosts an extreme flux of ionizing and far ultraviolet (FUV) photons. Proto-planetary discs in the ionizing environment near O stars in the Trapezium cluster are known to experience photoevaporation [10] . The stars experience mass loss due to heating both by FUV and by Lyman limit photons [11] . The former heat the disc to ∼ 10 3 K, generating outflows at the sound speed of ∼ 3 km s −1 , corresponding to the escape velocity at a distance ∼ 100 AU ( m * / M ⊙ ) from the star. Well within this distance, the FUV-driven outflow is diminished, though not entirely quenched [12] . At the ∼ 10 AU and smaller distances of interest here and given the extreme ionizing environment, Lyman continuum (ionizing) photons dominate the outflow, generating a ∼ 10 4 K ionized outflow moving at the sound speed of ∼ 10 km s −1 . This speed matches the escape velocity at a distance of d esc ∼ 10 AU ( m * / M ⊙ ) from the star. Loss from smaller distances occurs at a reduced rate, but still generates a ∼ 10 km s −1 outflow by the time the gas reaches d esc . Which process—tidal stripping or photoevaporation—dominates mass loss from the disc? Currently, tidal stripping dominates the unbinding of mass from the star, and at large distances from the star, tidal stripping determines the ultimate fate of the gas. However, the outflow properties of the observed cloud are nevertheless currently determined by photoevaporation. This can be understood as follows. Gas at a distance d > d t from its host star is accelerated by the tidal potential to a relative speed of Δ v , as it moves of order its own distance away from its host star: , so that , with . For d=d t , . At the cloud's current separation from SgrA*, at the tidal radius, comparable to the wind outflow rate. Hence, the motion of tidally decoupled gas is dominated by the tidal field. At earlier times in the star's plunge, Δ v was smaller, meaning that wind gas flowed out of the tidal radius faster than tidally disrupted gas. Currently, near the disc edge, the dynamics of previously ejected gas are set by properties of the wind, while on the ∼ 100 AU scale of the cloud, tidal evolution overwhelms wind motions. Although the current mass disruption rate of the proto-planetary disc, , is larger than the wind outflow rate, , wind gas emitted at earlier times dominates the currently observed cloud. In the short time that the infalling star has spent in an enhanced tidal field with d t < d out , the disc has only had the opportunity to expand by a fraction of its ∼ 10 AU size. At d =8 AU, the time since d t = d along the infalling star's orbit is Δ t =3 yr for m * =0.3 M ⊙ . Decoupled material has travelled only ∼ Δ v Δ t ∼ 4 AU further from the host star in that time. 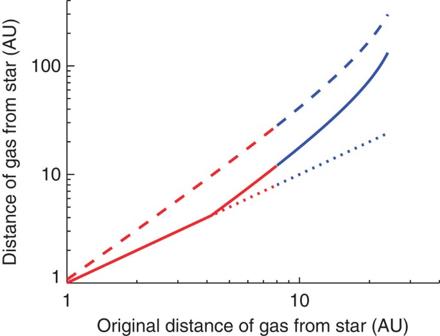Figure 2: Expansion of the infalling gas. As the star plunges towards the Galactic centre, its disc and the surrounding photoevaporative wind are tidally disrupted. For a fiducial stellar mass of, we plot the distance,d, of gas from the host star at the current epoch (solid line) and at the time of pericentre passage (dashed line) as a function of separation from the host star at the time of tidal decoupling. The dotted line represents no change. We assume that the material is instantaneously decoupled from the star when its separation equals the tidal radius and that it subsequently moves as a test particle in the gravitational field of the supermassive black hole. At the time of its decoupling, the test particle is started with the orbital parameters that the cloud had at timed/v*before decoupling, and the full separation between the test particle and the star is thereafter calculated as a function of time. Red portions of the curve represent gas initially in the disc, whereas blue portions represent gas initially in the photoevaporative cloud. For gas currently observed in the cloud, the tidal evolution depicted here dominates the wind structure at large scales, while the wind outflow at∼10 km s−1dominates the structure of recently ejected gas near the disc rim. At pericentre, tidal evolution determines the structure of the entire wind. Figure 2 illustrates this point. We ask how far a test particle, released at a given disc radius, d , from the star when d t = d and moving only under the gravity of the black hole, will be from its current orbit. Exterior to the decoupled material, gas originally launched in a wind dominates. Figure 2: Expansion of the infalling gas. As the star plunges towards the Galactic centre, its disc and the surrounding photoevaporative wind are tidally disrupted. For a fiducial stellar mass of , we plot the distance, d , of gas from the host star at the current epoch (solid line) and at the time of pericentre passage (dashed line) as a function of separation from the host star at the time of tidal decoupling. The dotted line represents no change. We assume that the material is instantaneously decoupled from the star when its separation equals the tidal radius and that it subsequently moves as a test particle in the gravitational field of the supermassive black hole. At the time of its decoupling, the test particle is started with the orbital parameters that the cloud had at time d / v * before decoupling, and the full separation between the test particle and the star is thereafter calculated as a function of time. Red portions of the curve represent gas initially in the disc, whereas blue portions represent gas initially in the photoevaporative cloud. For gas currently observed in the cloud, the tidal evolution depicted here dominates the wind structure at large scales, while the wind outflow at ∼ 10 km s −1 dominates the structure of recently ejected gas near the disc rim. At pericentre, tidal evolution determines the structure of the entire wind. Full size image The tidal decoupling rate in the disc is , where Σ( d ) is the original surface density of the disc and at the current position in the cloud's orbit. For illustration, we choose a profile similar to the minimum-mass solar nebula: Σ=Σ 0 ( d / d 0 ) −1 with Σ 0 =2×10 3 g cm −2 and d 0 =1 AU (ref. 5 ). This choice yields a current , where we set d equal to the current tidal radius. Photoevaporation, on the other hand, gives mass loss rates [13] , [14] of yr −1 for discs with sizes d out > d esc , where Φ i,49 is the ionizing luminosity, Φ i , in units of 10 49 s −1 of a source at distance D from the disc, with D pc = D /(1 pc). The photoevaporation mass loss can be derived as follows. At d = d esc , the escape velocity is comparable to the wind's sound speed c s =10 km s −1 . For d ≳ d esc , , where m p is the mass of a proton and we have neglected an order unity correction arising from the non-sphericity of the flow. We refer to the surface layer of the disc within which photoionization heats disc gas to ∼ 10 4 K as the 'base of the wind.' At the base of the wind, a balance between photoionization and radiative recombination yields a number density of , where α rec =2.6×10 −13 cm 3 s −1 is the Case B radiative recombination coefficient for hydrogen at a temperature of 10 4 K, and we have used the fact that the optical depth to ionizing photons is unity. Hence, . Though this expression is only good to order of magnitude, its coefficient is in fortuitously good agreement with more detailed wind models [13] , [14] . Observations yield 10 50.8 s −1 Lyman continuum photons in the central parsec [1] , [15] , corresponding to Φ i,49 =63. Using D =1 pc, . The central concentration of S-stars within 0.01 pc, which we estimate to contribute Φ i,49 =0.2 from each of ten approximately 10 M ⊙ stars comparable to the second-most luminous Trapezium star [13] , yields a small total of Φ i,49 =2 but in a more concentrated region. At the current position of the cloud, these stars contribute for D =6×10 −3 pc. At D =0.04 pc, this number is 35. For d =10 AU and smaller, mass loss from these ionizing fluxes dominates over FUV-driven mass loss. Using an intermediate value of . On the cloud's original orbit, , allowing our nominal disc, which contains ∼ 10 −2 M ⊙ between 1 and 8 AU, to survive for ∼ 10 6 yr. Disc masses several times larger are plausible, and hence a proto-planetary disc could have survived until the current time on the star's birth orbit in the ring. Dynamics of stripped gas Currently, gas farther than ∼ 12 AU from the star (for m * =0.3 M ⊙ ; see Fig. 2 ) was originally ejected in the photoevaporative wind. This ejected material (which starts in a ring-like configuration) itself undergoes tidal stripping. Along the star's original orbit, the extent of the wind moving at ∼ 10 km s −1 is set by the original 24 AU tidal radius. As gas requires only 10 years to travel 24 AU at ∼ 10 km s −1 , this wind scale applies even if the wind region was disrupted by close stellar encounters or more distant encounters with the black hole at some point in the past. As the star plunges towards the Galactic centre, its disc and wind are pulled off in shells as the tidal radius shrinks ( Fig. 3 ). The time for a parcel of wind to travel at 10 km s −1 from 10 to 100 AU is comparable to the 70-yr time to plunge to pericentre on the cloud's current orbit. This wind-generated cloud in turn experiences tidal disruption. By its current location, the original wind cloud will have reached an extent of a few hundred AU. Figure 2 illustrates this extent for . We note that although previous close encounters with the black hole may have stripped the disc to smaller than its original size, the disc wind is regenerated over each orbit. As long as the disc size exceeds d esc and most of the disc mass remains intact, our wind calculation remains valid. If the disc is stripped to smaller sizes, a wind will still be blown, but with reduced . 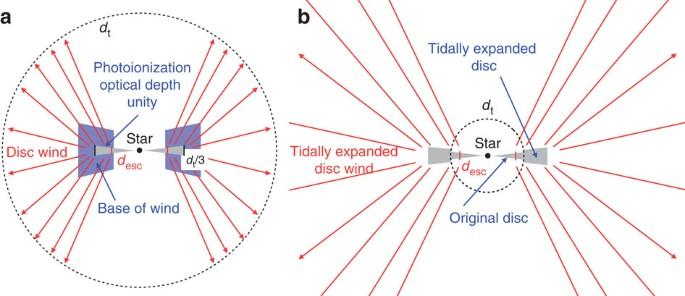Figure 3: Disc and wind structure. Schematic diagram of the disc and wind structure on the star's original orbit in the young stellar ring (a) and at the current epoch (b). On its original orbit, the star (black circle) hosts a protoplanetary disc (grey), which is limited in extent (vertical black line) to approximately one-third of the star's tidal radius,dt(dashed circle). Photoionization efficiently launches a wind beyonddesc, where gas is heated enough that its thermal velocity is comparable to the stellar escape velocity (vertical red line). From the wind-launching region (blue), gas flows outward (red arrows) until it passes the tidal radius and is stripped from the star. At the current epoch,dthas shrunk, causing both the disc and the wind to tidally expand. Figure 3: Disc and wind structure. Schematic diagram of the disc and wind structure on the star's original orbit in the young stellar ring ( a ) and at the current epoch ( b ). On its original orbit, the star (black circle) hosts a protoplanetary disc (grey), which is limited in extent (vertical black line) to approximately one-third of the star's tidal radius, d t (dashed circle). Photoionization efficiently launches a wind beyond d esc , where gas is heated enough that its thermal velocity is comparable to the stellar escape velocity (vertical red line). From the wind-launching region (blue), gas flows outward (red arrows) until it passes the tidal radius and is stripped from the star. At the current epoch, d t has shrunk, causing both the disc and the wind to tidally expand. Full size image Ram pressure of the ambient gas exceeds the ram pressure of the photoevaporative wind when , where n amb is the ambient number density of gas and v * is the star's velocity along its orbit. The characteristic density of ambient gas within the central 1.5 pc is n amb ∼ 10 3 cm −3 (ref. 16 ). Models place the density at ∼ 3×10 2 –6×10 3 cm −3 at the cloud's current location and ∼ (1–5)×10 2 cm −3 on its original orbit [17] . Along the star's original orbit, , and the ram pressure force from the disc wind roughly balances ram pressure with the ambient medium at the star's tidal radius. Currently, , so ram pressure with the surrounding medium has increased by 1–2 orders of magnitude at comparable separations from the star, and the tidally disrupted photoevaporative wind is undergoing ram pressure stripping. Nevertheless, at the current tidal radius, the two pressures remain in rough balance and our estimates of the mass loss rate are therefore valid. As the cloud continues its plunge towards the super-massive black hole, its outer (tidally detached) extent will be shaped by ram pressure stripping. 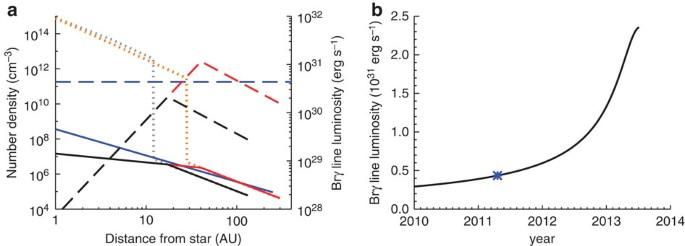Figure 4: Observational predictions. Ionized gas in the disc wind generates Brγ line luminosities in good agreement with observations. (a) Left axis: the cloud's ionized gas number density is inferred from the observed Brγ line luminosity to be1cm−3for emission dominated by gas at a distancedfrom the centre of the cloud (blue, solid). We approximate the neutral number density in the disc as, wherediis the initial separation of the gas from the host star and we use a disc scale heighthd∼0.1d. We show the ionized density,n+at the current epoch (black, solid) and at the time of pericentre passage (red, solid) for. Where wind gas dominates, we estimatewith, assuming that the wind geometry is not yet spherically symmetric. We choosedoutto be the current outer limit of the tidally disrupting disc. This estimate is not good at the largest separations, where tidal evolution and ram pressure stripping modify the gas density (see text). Where the disc itself is present, the neutral gas number density in the disc (grey dotted, current; orange dotted, pericentre) is 5–8 orders of magnitude larger than the ionized number density at the disc surface. We therefore setn+=nb, the number density at the base of the ionized wind (see text). Near the outer edge of the disc, the observed number density is in excellent agreement with the modelled density, given the approximate nature of this model. (a) Right axis: Brγ luminosity as a function of distance,d, from the infalling star, calculated using(in c.g.s. units) now (black, dashed) and at pericentre (red, dashed) for the same model. The currently measured line luminosity is included for reference (blue, dashed), and is in good agreement with the model. Most of the total integrated line emission is coming from near the current disc edge at 10–20 AU, but∼1/5 of the emission comes from∼100 AU scales. (b) Total Brγ line luminosity integrated over our model disc plus wind as a function of time, calculated as(in c.g.s. units; using 2πto adjust for a non-spherical wind). We predict that the total line luminosity will increase by approximately a factor of 5 from its reported value (blue asterisk) as the star approaches pericentre in 2013. Figure 4a displays the inferred ionized density of the cloud as a function of radial scale. From the total Brγ line luminosity, the discovery paper [1] calculates an electron density of , in excellent agreement with our prediction. In Fig. 4a , we also plot the contribution to the total line luminosity as a function of radial scale. As the luminosity is proportional to n 2 d 3 , this contribution peaks at the outer edge of the disc, but the contribution from the extended cloud falls off slowly, as 1/ d , so that about 1/5 of the line luminosity comes from 100 AU scales. We note that though the majority of Brγ emission comes from the 10–20 AU scale of the tidally expanded disc, the majority of the mass in the cloud is at large scales, as the cloud mass is proportional to nd 3 ∝ d . At these large scales, full hydrodynamic simulations including ram pressure stripping and tidal gravity in 3D are required to match in detail the surface brightness, shape and velocity width of the observed emission. One might naively expect the surface of the cloud to be Kelvin–Helmholtz unstable [1] . However, observations of cold fronts in X-ray clusters indicate that gas clouds moving at a Mach number of order unity through a hot ( ∼ keV) ambient medium maintain a smooth surface, probably owing to 'magnetic draping' [18] . Figure 4: Observational predictions. Ionized gas in the disc wind generates Brγ line luminosities in good agreement with observations. ( a ) Left axis: the cloud's ionized gas number density is inferred from the observed Brγ line luminosity to be [1] cm −3 for emission dominated by gas at a distance d from the centre of the cloud (blue, solid). We approximate the neutral number density in the disc as , where d i is the initial separation of the gas from the host star and we use a disc scale height h d ∼ 0.1 d . We show the ionized density, n + at the current epoch (black, solid) and at the time of pericentre passage (red, solid) for . Where wind gas dominates, we estimate with , assuming that the wind geometry is not yet spherically symmetric. We choose d out to be the current outer limit of the tidally disrupting disc. This estimate is not good at the largest separations, where tidal evolution and ram pressure stripping modify the gas density (see text). Where the disc itself is present, the neutral gas number density in the disc (grey dotted, current; orange dotted, pericentre) is 5–8 orders of magnitude larger than the ionized number density at the disc surface. We therefore set n + = n b , the number density at the base of the ionized wind (see text). Near the outer edge of the disc, the observed number density is in excellent agreement with the modelled density, given the approximate nature of this model. ( a ) Right axis: Brγ luminosity as a function of distance, d , from the infalling star, calculated using (in c.g.s. units) now (black, dashed) and at pericentre (red, dashed) for the same model. The currently measured line luminosity is included for reference (blue, dashed), and is in good agreement with the model. Most of the total integrated line emission is coming from near the current disc edge at 10–20 AU, but ∼ 1/5 of the emission comes from ∼ 100 AU scales. ( b ) Total Brγ line luminosity integrated over our model disc plus wind as a function of time, calculated as (in c.g.s. units; using 2 π to adjust for a non-spherical wind). We predict that the total line luminosity will increase by approximately a factor of 5 from its reported value (blue asterisk) as the star approaches pericentre in 2013. Full size image We predict ( Fig. 4b ) that the total Brγ luminosity of the cloud will increase as it approaches pericentre. This future evolution of a debris cloud around a low-mass star on a Keplerian orbit is easily distinguishable from that of a pressure-confined cloud with no self gravity or central mass supply. We further predict that with better resolution, the specific intensity of the line should increase, as most of the emission is coming from a smaller spread in velocities than is currently resolved. The dust in the wind, in analogy to dust in HII regions, does not reach temperature equilibrium with the 10 4 K gas. Gillessen et al . [1] argue that the dust continuum emission at about 550 K comes from small, transiently heated grains, having a total mass equal to ∼ 10 −5 the total gas mass of the cloud. Additional colder dust may be present. This relatively small dust mass may result from grain growth and settling in the proto-planetary disc, leaving relatively few small grains available to be lofted into the photoevaporative wind. The neutral, cooler disc does not contribute substantially to the observed dust emission. As demonstrated above, a disc can survive on the star's original orbit for ∼ 3 Myr. In the Supplementary Discussion , we discuss the likely rate at which such discs could be scattered onto orbits comparable to the observed gas cloud. This rate primarily depends on the highest mass scatterers in the ring of young stars around SgrA*. It could increase considerably above a minimum value 0.1% if the stellar mass function extends above the observed limit (as observed elsewhere in the galaxy), if there are intermediate mass black holes [19] of , or if compact star clusters (such as the observed clusters IRS 13N or IRS 13E) act as massive scatterers. Finally, if a 0.03 disc is disrupted by the black hole every ∼ 5 × 10 5 yr, the related events deliver to the inner 0.01 pc around SgrA*, comparable to the presently inferred accretion rate onto the black hole [20] . We note that alternative explanations invoking mass loss during rare evolutionary phases of stars (such as a proto-planetary nebula around an emerging white dwarf or a debris envelope around a merged blue straggler), have a much lower probability of occurance than our scenario. They share the requirement for a rare kick, but involve progenitors that are much less abundant than low-mass stars in the ring of young stars around SgrA*. The existence of proto-planetary discs in galactic nuclei has important implications: it could lead to a fragmentation cascade to comets, asteroids and dust around quasars [21] , and to bright flares due to the tidal disruption of planets [22] , as well as transits of hypervelocity stars [23] . In the Milky Way centre, the debris of proto-planetary discs offers a new probe of the low-mass end of the mass distribution of stars that are too faint to be detected otherwise. How to cite this article: Murray-Clay, R.A. & Loeb, A. Disruption of a proto-planetary disc by the black hole at the milky way centre. Nat. Commun. 3:1049 doi: 10.1038/ncomms2044 (2012).